Difluoromethylation of (hetero)aryl chlorides with chlorodifluoromethane catalyzed by nickel Relatively low reactivity hinders using chlorodifluoromethane (ClCF 2 H) for general difluoromethylation with organic molecules, despite its availability as an inexpensive industrial chemical. To date, transformations of ClCF 2 H are very limited and most of them involve difluorocarbene intermediate. Here, we describe a strategy for difluoromethylation of aromatics through nickel-catalyzed cross-coupling of ClCF 2 H with readily accessible (hetero)aryl chlorides. The reaction proceeds under mild reaction conditions with high efficiency and features synthetic simplicity without preformation of arylmetals and broad substrate scope, including a variety of heteroaromatics and commercially available pharmaceuticals. The reliable practicability and scalability of the current nickel-catalyzed process has also been demonstrated by several 10-g scale reactions without loss of reaction efficiency. Preliminary mechanistic studies reveal that the reaction starts from the oxidative addition of aryl chlorides to Ni(0) and a difluoromethyl radical is involved in the reaction, providing a route for applications of ClCF 2 H in organic synthesis and related chemistry. Difluoromethylation of organic molecules using chlorodifluoromethane (ClCF 2 H), an inexpensive industrial raw material used for production of fluorinated polymers [1] , represents a cost-efficient and straightforward route to the synthesis of paramount important fluorinated compounds [2] , [3] , [4] , [5] , [6] , [7] , [8] , [9] , [10] , [11] , [12] . Its activation and transformation, however, is still of great challenge, due to the strong C–Cl bonding in this gaseous compound. Thus far, most transformation paths of ClCF 2 H involve the difluorocarbene intermediate. The difluorocarbene species formed through pyrolysis at high temperature or through dehydrochlorination under strong basic conditions has very limited synthetic applications: the former is only applied to produce tetrafluoroethylene (TFE) and related fluorinated polymers (e.g., Teflon) [1] , and the latter is used to prepare heteroatom-substituted difluoromethylated compounds [13] , [14] , [15] , [16] . Very recently, we have developed a palladium-catalyzed difluoromethylation of arylborons with ClCF 2 H, also via a difluorocarbene pathway (Fig. 1a ) [17] . This study has also demonstrated that the activation of ClCF 2 H by transition metal can be conducted under mild reaction conditions and thus has wide application potential. Fig. 1 Strategies in activation of ClCF 2 H. a Previous work, activation of ClCF 2 H via a difluorocarbene pathway. b This work, a new activation of ClCF 2 H through a difluoromethyl radical pathway Full size image For both the practical application and the fundamental research, replacing the palladium catalyst by a first-row-based transition metal catalyst would pave a new and more cost-efficient way for applications of ClCF 2 H in organic synthesis and medicinal chemistry. Instead of ClCF 2 H activation, only rare examples of nickel catalyzed difluoroalkylation have been reported for the cross-coupling of difluoroalkyl chloride (ClCF 2 CO 2 Et) with nucleophilic arylboronic acids, in which the C–Cl bond is activated by an ester group (CO 2 Et) adjacent to the difluorocarbon [18] , [19] , [20] . As an inert substrate, the direct cleavage of C–Cl bond in ClCF 2 H remains a great challenge. Herein, we report a nickel-catalyzed reductive cross-coupling between ClCF 2 H and aryl chlorides [21] , [22] , [23] , [24] , [25] , [26] , [27] , representing an alternative strategy for the fluoroalkylation reactions. The reaction proceeds under mild reaction conditions with high efficiency and enables difluoromethylation of a variety of inexpensive and readily accessible aryl chlorides, including heteroaromatics and commercially available pharmaceuticals. The reaction can also extend to aryl bromides. In contrast to the difluorocarbene intermediate involved in the previous palladium-catalyzed process, the current Ni-catalyzed difluoromethylations undergoes a difluoromethyl radical pathway through the direct cleavage of C–Cl bond in ClCF 2 H. Optimization of the Ni-catalyzed cross-coupling We began our studies on nickel-catalyzed reductive cross-coupling between ClCF 2 H and aryl chlorides (Fig. 1b ). The use of aryl chlorides is because of their cheapness, ready availability, and more importantly, we proposed a direct transformation that can avoid the need for preformed arylmetals, such as arylborons and arylzincs. A suitable nickel catalytic system is the key to realize this synthesis route. To date, however, such a nickel catalyzed reductive cross-coupling between organohalides and fluoroalkylated electrophiles has not been reported and remains a challenge, because of the difficulties in selectively controlling the catalytic cycle to suppress the side reactions, such as the formation of hydrodehalogenated and dimerized fluorinated by-products. Although important progresses have been achieved in nickel-catalyzed reductive cross-coupling between aryl halides and unactivated alkyl halides [28] , [29] , specific challenges still exist in similar reactions of inert aryl chlorides without substitution by electron-withdrawing groups [30] , which is subject to the coupling reaction in the current study. 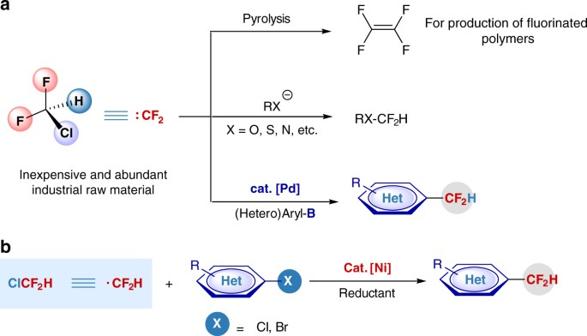Fig. 1 Strategies in activation of ClCF2H.aPrevious work, activation of ClCF2H via a difluorocarbene pathway.bThis work, a new activation of ClCF2H through a difluoromethyl radical pathway Accordingly, 1-( tert -butyl)-4-chlorobenzene 2a was chosen as the model substrate for this nickel-catalyzed difluoromethylation reaction (Table 1 ). Without additives, either no reaction or low yields of difluoromethylated arene 3a were observed in most of the experiments. The addition of MgCl 2 [31] (1.5 equiv.) benefited the reaction with 16% yield of 3a obtained when the reaction was carried out with NiCl 2 ·DME (10 mol%, DME, dimethoxyethane), bpy L1 (10 mol%, bpy, 2,2′-bipyridine) and Zn (2.0 equiv.) in DMA (dimethylacetamide) at 80 °C (entry 1). But other additives, such as HCl, TMSCl (trimethyl chlorosilane), or DIBAL-H (diisobutyl aluminum hydride) showed no reactivities (Supplementary Table 13 ). Encouraged by this result, a survey of the reaction parameters, such as ligands, nickel sources, and solvents, was conducted. Unfortunately, no significant improvement of the reaction efficiency was observed (entries 2–4 and Supplementary Tables 1 – 2 ). Since a more electron-rich nickel center can benefit the oxidative addition to C–Cl bond, the combination of two electron rich ligands L4 and DMAP (4-dimethylaminopyridine) [32] , [33] provided 3a in 46% yield (entry 5). Other pyridine-based ligands were also examined, but were inferior to DMAP (entries 6–8). Decreasing the reaction temperature to 60 °C with 10 mol% of NiCl 2 could improve the yield of 3a to 59% (entry 9). Further optimization of the reaction conditions (Supplementary Tables 4 – 12 ) revealed that the addition of 3 Å molecular sieves (MS) in conjunction with NiCl 2 (15 mol%) and L4 (10 mol%) could afford 3a in 79% yield (entry 10). In parallel, NiBr 2 as an alternative catalyst under the same reaction conditions could also lead to 3a in a comparable yield (entry 11). It should be mentioned that the use of 10 mol% of NiCl 2 and 10 mol% of L4 with 3 Å MS could also lead to 3a in a comparable yield (76%) sometimes. But in most of the cases, we obtained the yields of 3a in a range of 46% to 76%. We supposed that the use of excessive NiCl 2 vs L4 was probably because a comproportionation occurred between [Ni II ] and in situ generated [Ni 0 ]. Switching Zn with organic reductant tetrakis(dimethylamino)ethylene (TDAE) led to no 3a (Supplementary Table 14 ). The absence of nickel or L4 failed to provide 3a either (entries 12 and 13). Thus, these findings demonstrate that Ni/ L4 and Zn play an essential role in promotion of the reaction. 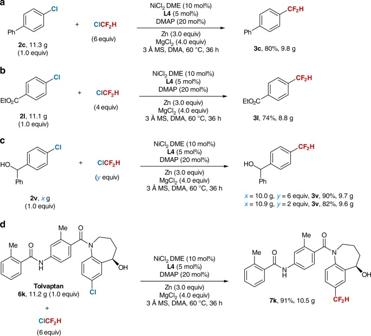Fig. 2 Ten-gram scale reaction of aryl chlorides with ClCF2H.aReaction of ClCF2H with2c.bReaction of ClCF2H with2l.cReaction of ClCF2H with2v.dReaction of ClCF2H with6k Table 1 Representative results for the optimization of Ni-catalyzed difluoromethylation of 2a with C1CF 2 H a Full size table Scope of the Ni-catalyzed cross-coupling With the viable reaction conditions in hand, a variety of aryl chlorides were examined (Table 2 ). For the electron-neutral aryl chlorides, the use of 10 mol% of NiCl 2 and L4 in a low amount as 5 mol% still provided corresponding difluoromethylated arenes in high yields ( 2b – 2d , 2x , and 2y ). Although the ortho substituted substrates, such as ortho methyl, fluoride, vinyl and ester substituted phenyl chlorides furnished the difluoromethylated products in lower yields ( 2e – 2g and 2n ), they are still synthetically useful for medicinal chemistry to access otherwise unavailable compounds. Aryl chlorides bearing electron-donating substituents were also amenable to the reaction, leading to 3h–3k in moderate to good yields ( 2h – 2k ), in which methoxyl group at meta position provided higher yield than that at para position ( 2i and 2h ). Thus, the current nickel-catalyzed process shows the much larger substrate scope than the previous nickel-catalyzed reductive cross-coupling, where the electron-rich and -neutral aryl chlorides have no reaction or only lead to poor yields [30] . Electron-deficient aryl chlorides were also competent coupling partners, highlighting the generality of this approach ( 2l – 2r ). The reaction exhibited good tolerance to functional groups including base or nucleophile-sensitive moieties, such as alkoxycarbonyl and enolizable ketone, and other groups such as vinyl, methylsulfonyl, nitrile, and substituted piperazine ( 2g , 2l–2t ). Remarkably, alcohol and arylboronate did not interfere with the reaction efficiency, and led to compounds 2u–2w in good yields, featuring the advantages of this approach. Furthermore, the reaction can also extend to aryl bromides, both electron-rich and electron-deficient aryl bromides were suitable substrates ( 2c′ , 2i′ , and 2l′ ). Table 2 Scope of the nickel-catalyzed reductive cross-coupling of ClCF 2 H with aryl chlorides a Full size table Synthesis of fluorinated heteroaromatic compounds is highly relevant to medicinal chemistry. To our delight, heteroaryl chlorides were also amenable to the current nickel-catalyzed reductive cross-coupling (Table 2 ). Pyridine-, quinoline-, and benzooxazole-containing substrates all underwent the reaction smoothly, leading to corresponding difluoromethylated heteroarenes in moderate to good yields ( 4a-4i ). 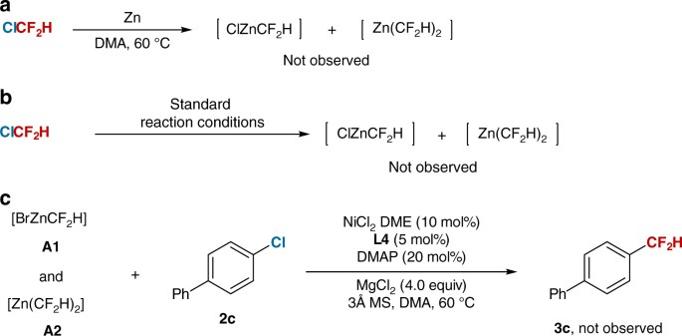Fig. 3 Reaction of ClCF2H with zinc.aReaction of ClCF2H with zinc in DMA.bReaction of ClCF2H with zinc under standard reaction conditions.cReaction of arylchloride2cwith difluoromethyl zinc species We also examined this protocol for direct difluoromethylation of aryl chloride containing pharmaceuticals, since difluoromethyl group is considered as a bioisostere of hydroxyl and thio groups, and also as a lipophilic hydrogen bond donor [34] , [35] (Table 3 ). Commercially available drugs such as fenofibrate, clofibrate, chlorodiphenhydramine and sibutramine underwent the current nickel-catalyzed process smoothly and afforded corresponding difluoromethylated products in good yields ( 6a – 6d ). The good tolerance of trialkyl amines of this coupling provides a useful route for the modulation of biologically active molecules. N -Heterocycles containing drugs were also viable in the reaction. For instance, clomipramine and buclizine furnished the desired products in good yields ( 6e and 6f ). Although lorcaserin bearing a free amine afforded low yield, the protected N -Boc-lorcaserin led to difluoromethylated arene efficiently ( 6g ). Furthermore, N -heteroaryl containing drug loratadine was also applicable to the cross-coupling and provided 7h in 82% yield ( 6h ). Most importantly, the acetyl protected empagliflozin, a drug used for the treatment of type II diabetes could also provide difluoromethylated product ( 6i) . Although only 25% yield of 7i was obtained, this strategy can trade off the yield for fast synthesis of various interesting new biologically active molecules in the late stage without the need for multi-step parallel synthesis. The rebamipide derivative with unprotected amide bond was also a competent coupling partner ( 6j ). This finding encouraged us to highlight the utility of this protocol further. As shown in 6k , the direct difluoromethylation of protic groups containing drug tolvaptan without protection of hydroxyl and amide bond produced corresponding difluoromethylated product in a yield as high as 92%. Thus, this protocol provides a synthetic simplicity route for the applications in drug discovery and development. Most remarkably, decreasing the loading amount of ClCF 2 H to 2 equiv. still provided difluoromethylated arenes with high efficiency as demonstrated by the synthesis of compounds 2a , 2h , 2l , 4f (Table 2 ), and 6k (Table 3 ), thus demonstrating the advantages of this approach. Table 3 Late-stage difluoromethylation of pharmaceuticals a Full size table To demonstrate the scalability of the current nickel-catalyzed process, several 10-g scale reactions of aryl chlorides were conducted. As shown in Fig. 2a , reaction of ClCF 2 H with 11.3 g of 4-chloro-1,1′-biphenyl 2c proceeded smoothly under standard reaction conditions, providing 3c in 80% yield. The electron-deficient aryl chloride 2l (11.1g) was also applicable to the reaction and afforded 3l even in a higher yield (74%) (Fig. 2b ). Notably, substrate bearing a hydroxyl group ( 2v ) could also furnish its corresponding difluoromethylated product 3v in a much higher yield (90%) (Fig. 2c ). Most remarkably, even 10-g scale late stage difluoromethylation of pharmaceutical tolvaptan 6k , a high yield (91%) was still obtained (Fig. 2d ). It is also worthy to note that decreasing the loading amount of ClCF 2 H to 2 equiv. could also lead to difluoromethylated arene without loss of reaction efficiency as shown by 10-g scale reaction of 2v (Fig. 2c ), thus demonstrating the good scalability and reliability of this reaction. In light of the wide existence of aryl chloride structural motif in pharmaceuticals and biologically active molecules, this approach would be useful in medicinal chemistry. Fig. 2 Ten-gram scale reaction of aryl chlorides with ClCF 2 H. a Reaction of ClCF 2 H with 2c . b Reaction of ClCF 2 H with 2l . c Reaction of ClCF 2 H with 2v . d Reaction of ClCF 2 H with 6k Full size image In the mechanism study of this reaction, we conducted several experiments. Firstly, to rule out the possible generation of difluoromethyl zinc species [10] , [11] in situ between ClCF 2 H and Zn, we performed control experiments. No difluoromethyl zinc species were observed in the reaction of ClCF 2 H with Zn in DMA at 60 °C, or even treatment of ClCF 2 H under standard reaction conditions in the absence of aryl chlorides (Fig. 3a, b ). Instead, only starting material ClCF 2 H was observed after the reaction. We also prepared difluoromethyl zinc species ( A1 and A2 ) by reaction of BrCF 2 H with Zn in DMA at 60 °C (Supplementary Methods) [36] ; however, no desired product 3c was obtained when these difluoromethyl zinc species were treated with aryl chloride 2c under standard reaction conditions (Fig. 3c ). Thus, these results exclude the pathway that the formation of difluoromethylated arenes is derived from the cross-coupling between difluoromethyl zinc species and aryl chlorides. On the basis of the previous reports [28] , [29] , we suggest that a nickel-based, reductive cross-coupling catalytic cycle is involved in the reaction. Fig. 3 Reaction of ClCF 2 H with zinc. a Reaction of ClCF 2 H with zinc in DMA. b Reaction of ClCF 2 H with zinc under standard reaction conditions. c Reaction of arylchloride 2c with difluoromethyl zinc species Full size image Secondly, to identify the initiation of current reaction from aryl chloride or ClCF 2 H, we prepared aryl nickel complex [ p - t Bu-PhNi(di t BuBpy)Cl] ( B1 ) [37] and difluoromethyl nickel complex [HCF 2 Ni(di t BuBpy)HCF 2 CO 2 ] ( C1 ) [38] , [39] . The structure of C1 was confirmed by X-ray crystallographic analysis (Fig. 4d ). To the best of our knowledge, the preparation of difluoromethyl nickel(II) complex has not been reported so far. The use of 4,4′-di t Bu-Bpy ( L2 ) instead of 4,4′-diNH 2 -Bpy ( L4) is because of the difficulties in isolation of [Ar-Ni( L4 )-Cl] and [CF 2 H-Ni( L4 )-HCF 2 CO 2 ]. In addition, L2 could also promote the reaction under standard reaction conditions and provided 3a in 39% yield (Fig. 4b ). A 15% yield of 3a was provided when B1 was treated with ClCF 2 H under standard reaction conditions (Fig. 4a ). Complex B1 could also serve as a precatalyst and provided 3a in 43% yield, which is comparable with the yield obtained by using NiCl 2 /di t BuBpy catalytic system (Fig. 4b ). However, no 3a was obtained by reaction of difluoromethyl nickel complex C1 with aryl chloride 2a (Fig. 4c ), demonstrating that the current reaction is initiated from aryl chloride and the possibility that the reaction starts from the oxidative addition of ClCF 2 H to Ni(0) is unlikely. Fig. 4 Mechanistic studies. a Reaction of nickel complex B1 with ClCF 2 H. b B1 or NiCl 2 /di t BuBpy catalyzed reaction of 2a with ClCF 2 H. c Reaction of C1 with 2a . d X-ray crystal structure of C1 . e Experiments to trap the difluoromethyl radical by reaction of 2c and 8 with ClCF 2 H. f Reaction of B1 and 8 with ClCF 2 H. g Reaction of 2a and 8 with C1 Full size image We also performed control experiments to gain some mechanistic insights into the reaction further (Fig. 4a ). The omission of Zn led to 3a in only 4% yield, implying that an active, low-valent nickel species is needed to promote the catalytic cycle by reduction of Ar-Ni II ( B1 ) with Zn. Inspired by the previous report, in which a reduction of Ar-Ni II to Ar-Ni I by reducing metals was proposed in the nickel-catalyzed coupling of aryl chlorides [40] , we envisioned that similar pathway may be involved in the reaction. Furthermore, a lower yield (11%) of 3a was provided without MgCl 2 (Fig. 4a ), indicating that the presence of MgCl 2 in current nickel-catalyzed process is probably to facilitate the reduction of nickel(II) complex by Zn to generate active nickel species. However, the exact role of MgCl 2 remains elusive. On the other hand, the omission of Zn/MgCl 2 could provide 3a in 12% yield (Fig. 4a ), suggesting that intermediate B1 reduction is not needed without MgCl 2 . Thirdly, to probe whether a difluoromethyl radical existed in the reaction, several radical trapping experiments were conducted. Radical inhibition experiments showed that the reaction could be readily inhibited by addition of electron transfer scavenger 1,4-dinitrobenzene [22] or a radical scavenger 2,2,6,6-tetramethyl-1-piperidinyloxy (TEMPO) (Supplementary Table 16 ). In addition, radical clock experiment showed that a ring-expanded product 9 was formed in 18% yield when ClCF 2 H was treated with α-cyclopropylstyrene 8 in the presence of aryl chloride 2c under standard reaction conditions (Fig. 4e ). However, when a radical scavenger TEMPO was added to the reaction, the reaction was totally inhibited without observation of compounds 9 and 3c (Supplementary Methods). Compound 9 could also be obtained by a stoichiometric reaction of nickel complex B1 with ClCF 2 H and 8 under standard reaction conditions (Fig. 4f ). But difluoromethyl nickel complex C1 failed to provide compound 9 (Fig. 4g ), thus ruling out the possible formation of compound 9 from C1 through the Ni-concerted insertion mechanism (Supplementary Fig. 142b ). Furthermore, the possibility of formation of compound 9 from aryldifluoromethyl nickel complex Ar-[Ni]-CF 2 H generated in situ between B1 and ClCF 2 H is also unlikely, as no ring-opening product 10 was observed by treatment of B1 with ClCF 2 H and 8 (Fig. 4f and Supplementary Fig. 142c ). Therefore, these results suggest that the formation of 9 via a radical pathway (Supplementary Fig. 142a ) is reasonable and a difluoromethyl radical species is involved in current catalytic cycle. Finally, to establish the role of DMAP in the reaction, we prepared nickel complexes [NiCl 2 (di t BuBpy)] ( D1 ) and [NiCl 2 (DMAP) 4 ] ( D2 ) [27] . Both of them could serve as precatalysts and provided 3a in comparable yields (Fig. 5a, b ). However, D1 provided 3a in a lower yield (16%) without DMAP (Fig. 5a ) and no 3a was observed by using D2 in the absence of di t BuBpy (Fig. 5b ). Additionally, a DMAP coordinated nickel complex B2 was observed by reaction of B1 with DMAP, which could also produce 3a in a 15% yield (Fig. 5c ). But only 6% yield of 3a was obtained without DMAP (Fig. 5d ). These results demonstrate that DMAP can function as a co-ligand to coordinate to the nickel center and thus facilitate the catalytic cycle. Fig. 5 The role of DMAP. a [NiCl 2 (di t BuBpy)] ( D1 ) catalyzed reaction between 2a and 1 with or without DMAP. b [NiCl 2 (DMAP) 4 ] ( D2 ) catalyzed reaction between 2a and 1 with or without di t BuBpy. c Reaction of B1 with ClCF 2 H in the presence of DMAP. d Reaction of B1 with ClCF 2 H without DMAP Full size image We also performed a Hammett-type analysis of the reaction (Supplementary Fig. 137 and 138 ). Plots of log( k rel ) versus σ and σ (−) were linear with moderate quality ( R 2 ∼ 0.93), and the slope ( ρ ) was between 1.9 and 2.0 [30] , [41] , [42] . The ρ values are smaller than those reports on stoichiometric studies of the oxidative addition of aryl halides to Ni (4.4–8.8) [43] , [44] , indicating that the oxidative addition of aryl chlorides to Ni(0) is not rate-determining step [45] . On the basis of these results and previous reports [28] , [29] , we propose that the reaction starts from aryl chloride via a radical-cage-rebound process [29] (Fig. 6a ). An oxidative addition of aryl chloride to Ni(0) initiates the reaction. Subsequently, the resulting nickel(II) complex [Ar-Ni II -Cl] ( B ) is reduced by Zn to generate [Ar-Ni I ] ( E ). E undergoes the second oxidative addition with ClCF 2 H to produce [Ar-Ni III -CF 2 H] ( F ) through a cage rebound process, in which a difluoromethyl radical ·CF 2 H is produced via a single-electron-transfer pathway, subsequently, the resulting ·CF 2 H rapidly recombines with [Ar-Ni II -Cl] to give F . Finally, F undergoes reductive elimination to deliver difluoromethylated arenes and [Ni I ]. [Ni I ] is further reduced by Zn to regenerate [Ni 0 ]. Alternatively, a radical chain mechanism [28] , [46] is also possible (Fig. 6b ) as the intermediate B1 could also lead to difluoromethylated product without reduction by Zn (Fig. 4a ). In this pathway, the ·CF 2 H generated by reaction of [Ni I ] with ClCF 2 H diffuses to the solution to combine with [Ar-Ni II -Cl] B to produce F , which undergoes reductive elimination to give difluoromethylated product. Finally, the resulting [Ni II ] is reduced by Zn to regenerate [Ni 0 ] (Supplementary Fig. 144 ). Fig. 6 Proposed reaction mechanism. a Proposed mechanism via a radical-cage-rebound process. b Proposed mechanism via a radical chain process Full size image In conclusion, we have developed a practical nickel-catalyzed difluoromethylation of (hetero)aryl chlorides and bromides with abundant and inexpensive ClCF 2 H, representing a new strategy for fluoroalkylation reactions. The reaction proceeds under mild reaction conditions and can efficiently access a wide range of difluoromethylated (hetero)aromatics, including pharmaceuticals. Comparing to the previous difluoromethylation methods [3] , [4] , [5] , [6] , [7] , [8] , [9] , [10] , [11] , [12] , [17] , the current nickel-catalyzed process features several advantages, inexpensive ClCF 2 H and low-cost nickel catalyst; more accessible and cheaper aryl chlorides as well as no need for preformed arylmetals; broad substrate scope including a variety of heteroaromatics and pharmaceuticals; synthetic simplicity and convenience without prefunctionalization of drugs and biologically active molecules. Particularly, the ability of direct modulation of pharmaceuticals by using ClCF 2 H provides good opportunities to discover new medicinal agents. The additives MgCl 2 and DMAP are critical to the reaction efficiency and DMAP can serve as a co-ligand to facilitate the catalytic cycle. Preliminary mechanistic studies reveal that the reaction starts from the oxidative addition of aryl halides to Ni(0) and a difluoromethyl radical is involved in the reaction, which is in contrast to the previous difluorocarbene pathway, thus paving a new way for applications of ClCF 2 H in organic synthesis and related chemistry. General procedure for the nickel catalyzed cross-coupling To a 25 mL of Schlenk tube were added aryl chloride 2 , 4 , or 6 (0.2 mmol, 1.0 equiv. ), NiCl 2 (10 mol%), L4 (5 mol%), zinc dust (3.0 equiv. ), MgCl 2 (4.0 equiv. ), 3 Å MS (100 mg) and DMAP (20 mol%). The mixture was evacuated and backfilled with argon for three times, DMA (2 mL) and ClCF 2 H 1 (2.6 M in DMA, 1.3 mmol, 6.5 equiv.) were then added. The Schlenk tube was screw capped and put into a preheated oil bath (60 °C). 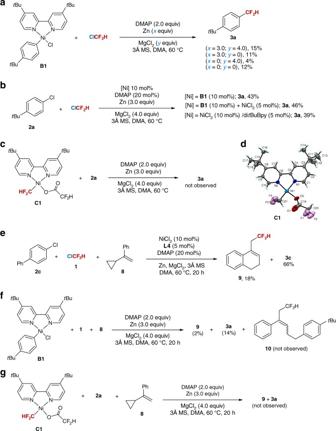Fig. 4 Mechanistic studies.aReaction of nickel complexB1with ClCF2H.b B1or NiCl2/ditBuBpy catalyzed reaction of2awith ClCF2H.cReaction ofC1with2a.dX-ray crystal structure ofC1.eExperiments to trap the difluoromethyl radical by reaction of2cand8with ClCF2H.fReaction ofB1and8with ClCF2H.gReaction of2aand8withC1 After stirring for 20 h, the reaction mixture was cooled to room temperature and diluted with ethyl acetate (2 mL). 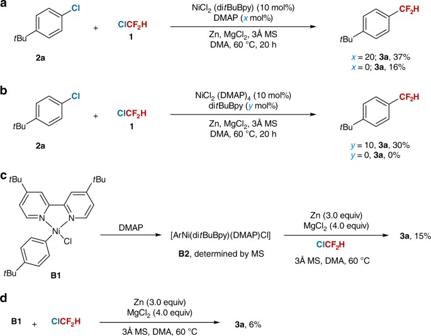Fig. 5 The role of DMAP.a[NiCl2(ditBuBpy)] (D1) catalyzed reaction between2aand1with or without DMAP.b[NiCl2(DMAP)4] (D2) catalyzed reaction between2aand1with or without ditBuBpy.cReaction ofB1with ClCF2H in the presence of DMAP.dReaction ofB1with ClCF2H without DMAP 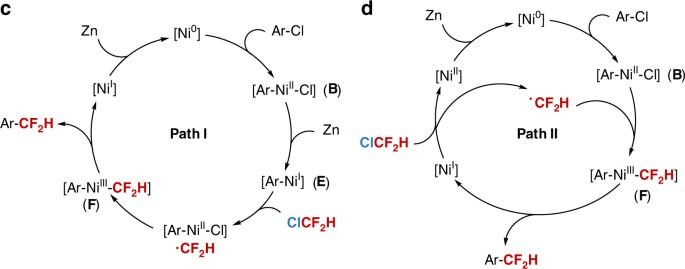Fig. 6 Proposed reaction mechanism.aProposed mechanism via a radical-cage-rebound process.bProposed mechanism via a radical chain process The yield was determined by 19 F NMR using fluorobenzene as an internal standard before working up. Then the reaction mixture was filtered with a pad of cellite. The filtrate was washed with brine, extracted with EtOAc for three times. Then the organic layer was dried over Na 2 SO 4 and concentrated. The residue was purified with silica gel chromatography to give product 3 , 5 , or 7 . Isolated yield is based on the average of two runs under identical conditions. Data availability The authors declare that all the data supporting the findings of this study are available within the paper and its supplementary information files. CCDC 1572871 contains the supplementary crystallographic data for C1 . These data can be obtained free of charge from the Cambridge Crystallographic Data Centre via www.ccdc.cam.ac.uk/data_request/cif .